Picosecond pulses from wavelength-swept continuous-wave Fourier domain mode-locked lasers Ultrafast lasers have a crucial function in many fields of science; however, up to now, high-energy pulses directly from compact, efficient and low-power semiconductor lasers are not available. Therefore, we introduce a new approach based on temporal compression of the continuous-wave, wavelength-swept output of Fourier domain mode-locked lasers, where a narrowband optical filter is tuned synchronously to the round-trip time of light in a kilometre-long laser cavity. So far, these rapidly swept lasers enabled orders-of-magnitude speed increase in optical coherence tomography. Here we report on the generation of ~60–70 ps pulses at 390 kHz repetition rate. As energy is stored optically in the long-fibre delay line and not as population inversion in the laser-gain medium, high-energy pulses can now be generated directly from a low-power, compact semiconductor-based oscillator. Our theory predicts subpicosecond pulses with this new technique in the future. Compact and reliable ultrashort pulse, high-energy laser sources [1] are of great importance for many fields in science and engineering, such as material processing, biomedical optics or optical communication. Compared with other gain media, the application of fully semiconductor-based laser sources can have many significant advantages owing to optimal compactness, robustness, cost-effectiveness, very-high wall-plug efficiency, simple current pumping, broadband gain bandwidth or spectral versatility. Since their first demonstration [2] , there has been great effort to improve the performance of ultrashort pulse generation with semiconductor lasers, reducing the pulse duration and increasing the output power [3] , [4] . Active-, passive- or colliding-pulse mode-locking techniques [5] , [6] were the prerequisite for the generation of few picosecond and subpicosecond pulses, considerably impeded due to non-linear phase changes associated with gain saturation [4] . So far, the shortest pulse durations from semiconductor lasers, reaching several tens of femtoseconds, have been demonstrated with optically pumped, passively mode-locked, vertical external-cavity surface emitting lasers (VECSELs) [7] based on wideband semiconductor saturable absorber mirrors [8] . However, a drawback of conventional mode-locked, q-switched or gain-switched semiconductor laser systems are the comparably low pulse energies as a direct consequence of the short carrier-relaxation time (~100 ps), high gain and low saturation energy in the semiconductor gain medium [4] , [5] , [9] . A major problem is that short carrier-relaxation times in the semiconductor gain media impede the realization of low repetition rate mode-locked systems. Thus, semiconductor lasers with higher pulse energies have very high levels of average output power, making them impracticable for many applications where compact, low-power light sources without extensive infrastructure are desired. In general, pulse energy can be increased using semiconductor-based master oscillator power amplifier systems. Whereas in case of single-spatial-mode semiconductor optical amplifiers (SOAs) the achievable pulse energies typically range from a few pJ to few tens of pJ [3] , [9] , higher energies become feasible using multispatial-mode semiconductor-based amplifiers like inverse bowtie SOAs [10] or tapered amplifiers [11] , [12] , [13] , [14] . Increased pulse energies can be achieved using the semiconductor-based eXtreme chirped pulse amplification concept [9] , where pulses are stretched temporally before amplification and the output energy of the recompressed pulse then exceeds the fundamental energy-storage limit of the semiconductor gain medium. Besides edge-emitting diodes, ultrashort pulses can be generated with optically pumped, passively mode-locked VECSELs [15] exhibiting increased saturation power and, thus, allowing for comparably high average output powers and pulse energies [16] . However, disadvantages of optical pumping can be, especially at high average power, a lower wall-plug efficiency and the need for a more sophisticated thermal management. In this work we introduce and investigate a fundamentally new concept of short-pulse generation based on Fourier domain mode-locked (FDML) lasers [17] , [18] , a recently introduced novel type of rapidly wavelength-swept lasers. Whereas picosecond or subpicosecond pulses with energies exceeding several nJ are hardly achievable with state-of-the-art semiconductor-based lasers and amplifiers, the FDML approach provides the potential for pulse energies reaching 100 nJ at repetition rates of several 100 kHz directly from the electrically pumped semiconductor-based oscillator. Fast wavelength-swept lasers with tuning rates of 0.1–1 MHz and sweep bandwidths of ~100 nm in the near infrared are the light sources of choice for today’s fastest optical coherence tomography (OCT) systems. OCT is a novel technique for high-resolution biomedical imaging, which finds widespread use from research set-ups to commercial systems already in clinical practice [19] , [20] , [21] . In standard wavelength-swept lasers, a narrowband optical filter is tuned over the gain spectrum of the laser medium. Lasing has to continuously build up from amplified spontaneous emission (ASE), causing a fundamental limit to the achievable sweep speed [22] . This limit can successfully be overcome using FDML lasers [17] , [18] , allowing for an up to 100-fold increase in sweep speed and, therefore, ultra-high OCT imaging speeds [23] . A main element of FDML lasers is the fibre delay line of ~1 km in the laser cavity, enabling the synchronization of the filter sweep frequency and the round-trip time of light in the cavity. This concept is similar to the one presented by Telle and Tang [24] . The ideal FDML laser is a semiconductor-based swept laser in a stationary operation mode, emitting periodic continuous-wave (cw) wavelength sweeps equivalent to highly chirped laser pulses. In this work we report for the first time on the optical compression of these sweeps, which is accomplished using a 15 km long, highly dispersive optical fibre. In this way we introduce a new approach of ultrashort pulse generation, with a very unique set of performance parameters regarding repetition rate and output pulse energy. The combination of low repetition rate, high pulse energy and high plug-wall efficiency might open access to many new applications. Standard mode-locked semiconductor-based lasers suffer from comparably low pulse energies because of the energy-storage limit in the semiconductor gain medium. However, FDML picosecond or subpicosecond pulses would have a unique advantage, as here the entire wavelength sweep with energies of up to 1 μJ is optically stored within the long delay fibre in the laser cavity and not as polulation inversion in the gain medium. Similar to eXtreme chirped pulse amplification concepts [9] , FDML lasers therefore have the potential to overcome this limit. Apart from high pulse energies, another advantage is that FDML lasers in principle enable direct access to the phase, that is, the chirp of the sweeps/pulses via control of the tunable bandpass filter and direct access to the amplitude by the current of the semiconductor gain medium. This means an FDML laser has a pulse shaper inherently built in. It should be emphasized that this method of ultrashort pulse generation is fundamentally different from conventional mode locking, such as the well-known soliton mode locking and stretched-pulse (dispersion-managed) solutions to the Haus master equation [25] , as well as the recently discovered all-normal-dispersion [26] , similariton [27] and soliton-similariton [28] regimes. Besides the fact that this concept might be an attractive candidate for future high-energy, low repetition rate semiconductor pulse lasers, our findings, that is, the measured compression factor, also provide valuable insight into the coherence of the FDML output. In this work we demonstrate that pulse duration very critically depends on the coherence properties of the FDML laser, currently allowing for temporal compression down to 60–70 ps. The experimental results are compared with numerical simulations based on a theoretical model of the FDML laser [29] . Simulations also enable us to give an outlook how pulse duration might significantly be improved in the future. Temporal compression of the FDML sweeps The FDML resonator in Fig. 1a uses a 1,550±50 nm SOA as gain medium and a bulk Fabry–Pérot tunable filter (BFP-TF) [23] with a finesse of ~400 for very-high sweep speeds of ν sweep ~250 nm μs −1 at 2 × 390 kHz repetition rate. The 524 m fibre delay line is dispersion compensated to improve the coherence of the laser [30] , [31] . Light from the FDML output passes a second, single polarization (16 dB polarization dependence) booster SOA, which ensures a stable polarization state and acts as an optical switch, only transmitting and amplifying a part of each forward (short to long wavelengths) sweep. This determines the temporal width of the sweep τ sweep , the sweep bandwidth Δ λ sweep and the centre wavelength λ c of the sweep used for temporal compression. Our optical compressor is a 15 km long dispersion compensation fibre (DCF), which is passed either once (‘1 × pass’) or four times (‘4 × pass’). To ensure optimum compression, the filter-drive parameters have to be chosen very accurately (see Methods). An additional chirp, which might be introduced by the rather slow ~18 ns switching of the SOA gain, should be very small and can, if necessary, be compensated by fine tuning of the filter-drive parameters (see Methods). For all measurements, a good polarization contrast is observed after the optical compressor. Fig. 1b shows the wavelength tuning of the bandpass filter for 1 × pass of the DCF (amplified part red). The pulses are analysed with a fast-sampling oscilloscope and a second-harmonic intensity autocorrelator. 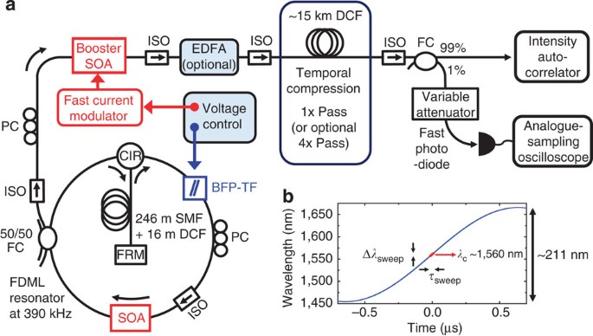Figure 1: Experimental set-up and bandpass filter control. (a) FDML resonator operated at 1,560 nm and 390 kHz repetition rate, post-amplification devices, DCF used for temporal compression and the detection system for the short pulses. ISO, optical isolator; PC, polarization controller; FRM, Faraday rotation mirror; CIR, optical circulator; FC, fused fibre coupler. (b) Typical wavelength tuning (1 × pass of DCF) of the optical bandpass filter (blue), including the part used for temporal compression (red). Figure 1: Experimental set-up and bandpass filter control. ( a ) FDML resonator operated at 1,560 nm and 390 kHz repetition rate, post-amplification devices, DCF used for temporal compression and the detection system for the short pulses. ISO, optical isolator; PC, polarization controller; FRM, Faraday rotation mirror; CIR, optical circulator; FC, fused fibre coupler. ( b ) Typical wavelength tuning (1 × pass of DCF) of the optical bandpass filter (blue), including the part used for temporal compression (red). 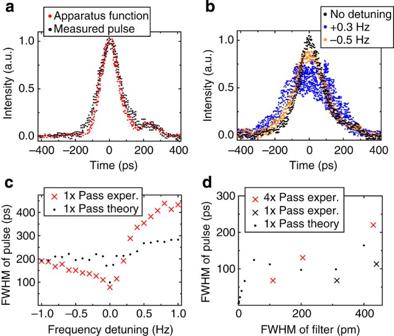Figure 2: Pulses from FDML laser. (a) Apparatus function of photodiode and oscilloscope, and the pulse generated from the compressed FDML sweep (1 × pass of DCF and bandwidth Δλsweep~6 nm). Deconvolution yieldsτpulse~68 ps. (b) Pulses from the FDML laser for different FDML frequency detunings. All illustrations showing pulses are based on digitized photographs of the analogue-sampling oscilloscope. (c) Degradation of pulse width (FWHM) for FDML frequency detuning (~3 × 10−7relative to drive frequency), showing measured values and results from theory. (d) Pulse width (FWHM) plotted against spectral width (FWHM) of the tunable bandpass filter, showing measured values in case of a 4 × pass and 1 × pass of the DCF fibre, and results from theory in case of 1 × pass of the DCF fibre. Full size image Internal FDML parameters and their impact on pulse duration Figure 2a shows the ~127±3 ps apparatus function of the sampling oscilloscope and photodiode, measured with pulses from a titanium sapphire laser (see Methods). Figure 2a also shows the signal from the shortest pulse (full width at half maximum (FWHM) ~144±3 ps). By numerical deconvolution, a duration of ~68±12 ps (assuming a Gaussian shape) can be estimated. The uncertainty of the pulse duration caused by electronic measurement and deconvolution was calculated from the fluctuations of the pulse duration on the sampling oscilloscope via error propagation methods (here ±12 ps). In this measurement, light passed the DCF once and the bandwidth Δ λ sweep is set to ~6 nm ( τ sweep ~24 ns) to reduce effects of higher-order dispersion in the DCF. Figure 2b show the pulse durations for frequency detunings ranging from −1 to 1 Hz. It is obvious that already a slight detuning of the FDML filter-drive frequency on the order of Δ f ~0.1 Hz (that is, a relative frequency change of ~3 × 10 −7 ) results in considerable temporal broadening of the pulses (increase of pulse duration by a factor of ~1.5). These values of detuning are far too small to significantly change the amount of dispersion required for compression. This shows that internal laser dynamics governs the output of the FDML sweep rather than only specifications of the individual components, for example, the sweep filter. As shown in Fig. 2c , the experimental values found with our set-up are in good agreement with numerical simulations using the theoretical model described in [29] and [32] , even though the discrepancy between theory and experiment reaches a factor of up to ~2. The deviation of the minimum value of the achievable pulse duration measured in the experiment to the minimum value predicted by theory is ~30%. However, the observed asymmetry for detuning is much less pronounced in the theory; only the trend is predicted qualitatively. To mimic experimental conditions (sampling oscilloscope) and suppress fluctuations, the theoretical pulse durations have been achieved by averaging the simulated intensity profiles of over 20 non-sequential pulses, evaluating every 100th round trip. In this way a variation of the pulse duration of up to ~20% is observed, depending on the chosen trigger condition for averaging, giving an idea of the uncertainty of the presented theoretical data. Figure 2: Pulses from FDML laser. ( a ) Apparatus function of photodiode and oscilloscope, and the pulse generated from the compressed FDML sweep (1 × pass of DCF and bandwidth Δ λ sweep ~6 nm). Deconvolution yields τ pulse ~68 ps. ( b ) Pulses from the FDML laser for different FDML frequency detunings. All illustrations showing pulses are based on digitized photographs of the analogue-sampling oscilloscope. ( c ) Degradation of pulse width (FWHM) for FDML frequency detuning (~3 × 10 −7 relative to drive frequency), showing measured values and results from theory. ( d ) Pulse width (FWHM) plotted against spectral width (FWHM) of the tunable bandpass filter, showing measured values in case of a 4 × pass and 1 × pass of the DCF fibre, and results from theory in case of 1 × pass of the DCF fibre. Full size image For a more systematic investigation, Fig. 2d shows the minimum achievable pulse duration τ pulse in case of different spectral widths Δ λ Filter of the BFP-TF for 1 × pass (Δ λ sweep ~6 nm, τ sweep ~24 ns, ν sweep ~250 nm μs −1 ) and 4 × pass (Δ λ sweep ~1.5 nm, τ sweep ~24 ns, ν sweep ~62.5 nm μs −1 ) of the DCF fibre compressor. With a fixed finesse of ~400 (mainly given by the coatings) the filter width Δ λ Filter can be adjusted by adapting the free spectral range (FSR) of the BFP-TF. Depending on Δ λ Filter , the FSR therefore ranges from ~40 to ~170 nm. The measurements indicate that τ pulse correlates to a certain extent with Δ λ Filter (smaller Δ λ Filter yields smaller τ pulse ), but also with ν sweep (larger ν sweep gives shorter τ pulse for same Δ λ Filter ). Currently, there are two different limits to the filter width Δ λ Filter accessible in the experiment: (1) For the case of 1 × pass of the DCF fibre compressor, Δ λ Filter was not reduced below ~315 pm, as the necessary further reduction of the FSR requires an increase in mechanical excursion of the BFP-TF, which is not possible owing to mechanical restrictions. (2) For the case of 4 × pass of the DCF fibre compressor, mechanical restrictions are currently not limiting. The 4 × pass generates 4 × more dispersion; hence, it can compensate a sweep/pulse with 4 × more chirp. A 4 × higher chirp of the sweep translates to a 4 × slower sweep speed of the FDML laser, reducing the mechanical requirements for the filter. Hence, in the case of 4 × pass we were not able to reduce Δ λ Filter below ~110 pm, because the centre wavelength λ c of the sweep does not coincide with the gain maximum and, therefore, smaller values of FSR induce lasing at wrong wavelengths. In the future, the application of a BFP-TF with higher finesse can enable considerably smaller filter widths Δ λ Filter . Currently, a minimum pulse duration τ pulse of ~68±12 ps has been achieved in both cases, that is, in case of 1 × pass and of 4 × pass. Intensity autocorrelation and continuum generation To confirm the electronic measurements with autocorrelation data, we applied erbium-doped fibre amplification (EDFA) to raise the power levels (1 × pass of DCF). To minimize non-linear effects and prevent pulse break-up, we limited our EDFA gain to ~16 dB, resulting in a pulse width τ pulse ~59±12 ps, measured with the sampling oscilloscope. 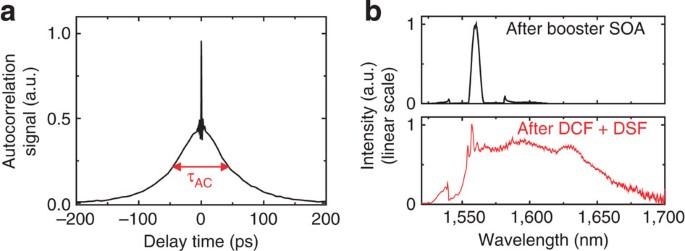Figure 3: Autocorrelation signal and continuum generation. (a) Background-free second-harmonic intensity autocorrelation signal of the amplified FDML pulse (1 × pass of DCF, Δλsweep~6 nm). A narrow coherence spike (time-bandwidth limit of ~600 fs) is centred on top of a broad pedestal (τAC~89 ps), implying a pulse width (FWHM)τpulse~63 ps. (b) Time-averaged spectrum after the booster SOA (top) and very flat continuum (linear scale) measured after ~15 km DCF and additional 1.7 km dispersion shifted fibre (DSF; bottom). (Small satellite peaks result from adjacent Fabry–Pérot modes, remaining after suppression by the booster SOA). Figure 3a shows the corresponding autocorrelation signal, which exhibits two features. A narrow coherence spike (consistent with the bandwidth limit of ~600 fs) is centred on top of a broad pedestal (FWHM, autocorrelation time τ AC ~89 ps; contrast ratio ~1:1). This implies a pulse width of τ pulse ~63 ps consistent with the results acquired with the sampling oscilloscope, but also indicates the existence of an intensity substructure [33] , [34] caused by internal FDML dynamics (see Discussion) [33] , [34] . Note that the uncertainty of the autocorrelation measurement itself can be considered negligible. However, the error caused by the unknown pulse shape can be estimated to be ~10 ps (Gaussian: 63 ps; Sinc 2 : 67 ps; Sech 2 : 58 ps). The average power and the instantaneous power after the DCF are ~2.2 mW and ~96 W, respectively. This corresponds to a pulse energy of ~5.6 nJ at a pulse repetition rate of 390 kHz. Figure 3b (top) shows the spectrum after the booster SOA, whereas Fig. 3b (bottom) demonstrates the potential of continuum generation, realized by propagation of the pulses (pulse energy ~11 nJ) through 1.7 km of dispersion shifted fibre. We observe remarkable spectral flatness over ~100 nm even on a linear scale. Although continua can even be generated with cw-sources, the extremely low average power of our source might be attractive in several configurations. Figure 3: Autocorrelation signal and continuum generation. ( a ) Background-free second-harmonic intensity autocorrelation signal of the amplified FDML pulse (1 × pass of DCF, Δ λ sweep ~6 nm). A narrow coherence spike (time-bandwidth limit of ~600 fs) is centred on top of a broad pedestal ( τ AC ~89 ps), implying a pulse width (FWHM) τ pulse ~63 ps. ( b ) Time-averaged spectrum after the booster SOA (top) and very flat continuum (linear scale) measured after ~15 km DCF and additional 1.7 km dispersion shifted fibre (DSF; bottom). (Small satellite peaks result from adjacent Fabry–Pérot modes, remaining after suppression by the booster SOA). Full size image From a laser physics point of view, the observed pulse duration τ pulse gives a direct indication of the degree of coherence in the FDML sweep. In case of a fully incoherent wavelength sweep, the shortest achievable pulse length τ inc for the compression is determined by the instantaneous linewidth Δ λ inst (refs 32 , 35 ) and the sweep speed ν sweep (see Methods), as sketched in Fig. 4a (dark green curve, 1 × pass; dark blue curve, 4 × pass). Temporal compression of a per se incoherent wavelength-swept ASE [36] , [37] with adjustable instantaneous linewidth [36] (see Methods) demonstrates very good agreement with this model (see crosses in Fig. 4a ). Assuming equal filter width, the minimum pulse lengths achieved with incoherent light are ~20 × longer than with FDML (compare achievable pulse durations for incoherent wavelength-swept ASE ( Fig. 4a ) and for FDML operation ( Fig. 2b )). In case of a fully coherent wavelength sweep with Δ λ sweep ~6 nm (1 × pass) or Δ λ sweep ~1.5 nm (4 × pass), the minimum achievable pulse durations τ coh are ~600 fs or ~2.4 ps (see Methods), respectively; both are considerably smaller than the ~68 ps achieved with FDML. This indicates that the FDML sweep has non-coherent contributions in its amplitude and phase evolution. However, a purely incoherent sweep can never generate a τ pulse of ~68 ps, as illustrated in Fig. 4b (only 4 × pass), as all values of the dark blue curve (expected pulse duration for incoherent sweep, see Methods) are at least ~5 × larger. On the basis of the measured instantaneous linewidth [31] , [35] (not filter width) of ~10 pm (see Methods), the red oval indicates the approximate operation range of the FDML laser, clearly located within the parameter range of partial coherence (yellow area). 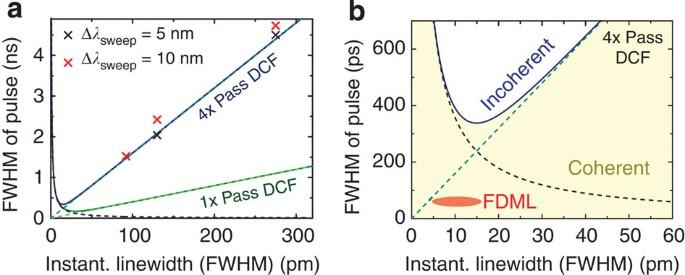Figure 4: Pulse duration for incoherent sweeps. (a) Pulse duration of the temporally compressed output of a wavelength-swept light source as function of the instantaneous linewidth Δλinst, assuming purely incoherent superposition (dark blue curve: 4 × pass, dark green curve: 1 × pass), each case defined by the convolution of two contributions: (i) time-bandwidth product of Δλinst(black dashed curve) and (ii) limitation due to sweep speed of the optical bandpass filter (blue dashed curve, 4 × pass; green dashed curve, 1 × pass). The crosses show the experimental results with an incoherent wavelength-swept ASE source for 4 × pass of DCF and different bandwidths Δλsweep. (b) Zoomed view, representing current FDML performance for 4 × pass of DCF (red oval), clearly lying within the partially coherent region (yellow area). Figure 4: Pulse duration for incoherent sweeps. ( a ) Pulse duration of the temporally compressed output of a wavelength-swept light source as function of the instantaneous linewidth Δ λ inst , assuming purely incoherent superposition (dark blue curve: 4 × pass, dark green curve: 1 × pass), each case defined by the convolution of two contributions: (i) time-bandwidth product of Δ λ inst (black dashed curve) and (ii) limitation due to sweep speed of the optical bandpass filter (blue dashed curve, 4 × pass; green dashed curve, 1 × pass). The crosses show the experimental results with an incoherent wavelength-swept ASE source for 4 × pass of DCF and different bandwidths Δ λ sweep . ( b ) Zoomed view, representing current FDML performance for 4 × pass of DCF (red oval), clearly lying within the partially coherent region (yellow area). Full size image Hence, the entire FDML sweep is at least partially or section-wise coherent. The question whether the electric field of the FDML sweep consists of many sections with internally high phase and amplitude stability, but random phases between each other, or if random phase and amplitude fluctuations have some increased probability near the optimum phase and amplitude evolution cannot be judged at this point with certainty. However, as we operate our FDML laser in the ultra-stable regime as observed by Kraetschmer et al. [38] , it can be speculated that the FDML sweeps show a section-wise very good coherence, interrupted by wavelength/phase discontinuities. This assumption is supported by the observation of interference fringe signals from a Mach–Zehnder interferometer, where sections of very smooth and clean fringe signals can be observed, separated by more unstable regions of phase discontinuities. After compression, the weakly defined phase between the different sections causes strong amplitude fluctuations, which have also been observed in the numerical simulations. To conclude, in this work we demonstrate for the first time the temporal compression of the wavelength-swept cw output of an FDML laser. Approximately 60–70 ps pulses at a repetition rate of 390 kHz have been achieved. Because of uncompensated higher-order chirp, only 6 nm sweep range has been used, which currently is the reason for limited pulse energies of ~140 pJ (without EDFA) and ~5.6 nJ (with EDFA). Concerning the achievable pulse energy, these results cannot compete with master oscillator fibre power amplifier systems [39] , but are comparable to semiconductor-based, optically pumped VECSELs [15] , [16] or semiconductor-based master oscillator power amplifier systems [12] , [14] . Nevertheless, it should be emphasized that in spite of current experimental restrictions, already the ~140 pJ is higher than typical pulse energies achievable with conventionally mode-locked SOA-based semiconductor lasers [9] , even in the case of using an eXtreme chirped pulse oscillator approach [40] . In the future, the additional application of chirped fibre Bragg gratings [30] for arbitrary dispersion compensation might make >100 nm sweep ranges usable, which would already push the pulse energy of the ~60–70 ps long pulses directly from this laser oscillator without an amplification well into the nJ range, even including compressor losses [30] . Moreover, the additional use of chirped fibre Bragg gratings could minimize non-linear effects in the optical compressor and, therefore, reduce or prevent the effect of pulse break-up limiting pulse energy. For example, if the final compression from nanoseconds to picoseconds is performed by a chirped fibre Bragg grating at the very end of the fibre set-up, the propagation length of the pulse at maximum peak power can be minimized. Alternatively, a final bulk optics compressor may be used. Using an EDFA, a pulse energy of more than 11 nJ is feasible tolerating degradation of pulse duration. This is sufficient for the generation of a spectrally flat continuum. The ~60–70 ps pulse duration is far shorter than the result expected from purely incoherent superposition, indicating, at least partially coherent superposition of the different spectral components of the FDML sweep during the compression process. The experiments are in good agreement with numerical simulations, which predict that <10 ps pulses can be achieved with the current set-up by simply using a more narrowband sweep filter (higher finesse). Remarkably, an even further reduction in pulse duration is predicted by theory, reaching almost bandwidth-limited pulses if, in addition to a more narrowband filter, the cavity dispersion is further reduced. These findings indicate that, in the future, modifications in the experiment will enable the generation of considerably shorter pulses well into the lower picosecond range. However, it should be emphasized that even the 60–70 ps pulse durations of our set-up presented here are highly attractive for many applications. Usually, picosecond pulses have a very narrow spectrum due to the time-bandwidth product; this makes them prone to parasitic, coherent, non-linear effects like Brillouin scattering [41] , which limits the maximum achievable pulse energy, especially in fibre-based delivery systems. Moreover, all applications that are susceptible to interference caused by spurious reflections greatly benefit from the wide spectral bandwidth. In imaging applications the wide spectrum reduces problems with speckle noise, whereas in sensing applications it reduces spectral modulations caused by back reflections. Considering the described potential for improvement, FDML lasers might become an interesting option as compact, all fibre-based and highly robust source for ultrashort pulses. Even though pulse energies from the FDML laser without EDFA currently do not reach the performance of state-of-the-art semiconductor-based pulse laser systems [9] , [15] , [16] , the low repetition rate of FDML lasers, the fact that they are constructed of all fibre-based low-cost telecom components and the fact that they are electrically pumped may make them highly attractive for applications that demand compactness, low power consumption and robust design. FDML laser resonator and booster SOA The optical delay line in the FDML resonator consists of a 246 m standard, single-mode fibre (Corning SMF 28) and a 16 m DCF (OFS-HFDK) used to minimize residual dispersion in the resonator in the wavelength range around 1,560 nm to less than 0.25 ps nm −1 . A σ-ring configuration is used with an optical circulator and a Faraday rotation mirror; hence, light passes the delay line twice during one resonator round trip and birefringence effects in the delay line are cancelled. The circulator and the optical isolator ensure unidirectional lasing. Fifty per cent of the optical power is coupled out via a fused fibre coupler. The gain of the SOA in the cavity is polarization-independent (Covega SOA1117), whereas the gain of the booster SOA is polarization-dependent (Covega BOA1004). Polarization controllers enable adjustment of the polarization state in the fibre. A two-channel, phase-locked voltage control is used. Channel 1 (DC+AC voltage) generates a sinusoidal wavelength tuning of the BFP-TF. The DC voltage is actively feedback-controlled to stabilize the centre wavelength λ c , using an optical spectrum analyser. Channel 2 yields a synchronous switching of the gain of the booster SOA via a fast current modulator (Wieserlabs WL-LDC10D). Light is either amplified from ~10 mW average power before the booster SOA to ~47 mW instantaneous power (SOA on) after the booster SOA or suppressed by >10 dB (SOA off). Temporal compression and filter-drive parameters The optical compressor is an ~15-km long, highly dispersive DCF fibre (OFS type HFDK). Light passes the fibre once (‘1 × pass’) or four times (‘4 × pass’). For all experiments, a centre wavelength of λ c =1,560 nm is chosen, as this is a good trade-off between large amount of negative dispersion (−4 ns nm −1 ) of the DCF, minimal loss (approximately −8.5 dB) and good dispersion compensation in the FDML resonator. The ~211 nm total-filter sweep range of the BFP-TF is set such that the filter sweep speed ν sweep ( λ c ) equals the inverse of the magnitude of the dispersion in the DCF compressor. To guarantee minimal loss, a very high sweep speed of the BFP-TF is crucial, as it minimizes the required DCF fibre length. However, some measurements are performed with light passing ~15 km of DCF fibre four times (two directions and two orthogonal polarizations) using an optical circulator and a polarization beam splitter. In this case, dispersion and loss are increased and the required total filter sweep range (~53 nm) is reduced by a factor of 4. Because of the dispersion slope of the DCF and the sinusoidal drive of the optical filter, there exists a limit for temporal compression τ com (Δ λ sweep ) caused by remaining higher-order dispersion, depending on the chosen bandwidth Δ λ sweep . Besides accurate adjustment of the total filter sweep range, a reasonable choice of the phase difference ΔΦ between filter-drive and booster SOA modulation signal is important, so the curvature of the drive can partly compensate the dispersion slope in the DCF. Simulations using the measured dispersion [42] of the DCF predict τ com <10 ps for an optical sweep bandwidth Δ λ sweep ~6 nm (1 × pass) and Δ λ sweep ~1.5 nm (4 × pass). Erbium-doped fibre amplification The EDFA used in this experiment consists of ~6 m of doped fibre (MetroGain M12-980-125) and two wavelength division multiplexers. Pump light from a pump diode (JDSU-S34) at 1,457 nm is used in forward direction. Benefiting from a small duty cycle (~1%), an amplification of the truncated sweep ( τ sweep ~24 ns, Δ λ ~6 nm) by at least 16 dB is easily possible. By far higher amplification factors can be achieved, but the spectral shape and the pulse duration degrade because of non-linear processes in the compression fibre. However, for our experiment the 16 dB amplification is sufficient to measure a second-harmonic intensity autocorrelation. Sampling oscilloscope and autocorrelator For measurement and characterization of the pulse duration, two methods are used. First, a direct electronic measurement using an 8-GHz photo receiver (Kyosemi Corporation KPDX10GV3) and an analogue-sampling oscilloscope (Tectronix 7603). Second, a home-built second-harmonic intensity autocorrelator. For the electronic measurement, 1% of the compressed light is adjusted in power by a bulk optic variable attenuator. To guarantee proper triggering of the sampling oscilloscope (~25 ps rise time), the train of pulses is split by a 50/50 fibre coupler; one part is directly used to trigger the oscilloscope (2 GHz photodiode (Wieserlabs WL-PD2GA)), the other part is optically delayed by a length of ~100 m single-mode fibre and measured with the fast photodiode. To determine the apparatus function of photodiode and oscilloscope, short pulses (several picoseconds) from the amplified output of a 74 MHz titanium sapphire oscillator (Femtolasers Integral, 975 nm part, post-amplified by Yb fibre amplifier—set-up described in [43] ) were measured in the same manner yielding an FWHM of ~127±3 ps. The home-built second-harmonic intensity autocorrelator for measurements up to 500 ps pulse length uses a BIBO crystal in a non-collinear geometry for frequency doubling, generating a background-free signal. The frequency-doubled signal is detected with an integrating silicon photodiode (Wieserlabs WL IPD4A) adjusted to 250 μs integration time and a read-out rate of ~900 Hz. Each data point is a 100 times average. Theoretical model of pulse duration after compression To gain a comprehensive understanding of pulse generation based on temporal compression of wavelength-swept waveforms, it is important to theoretically analyse the minimum achievable pulse duration for both limiting cases, assuming fully coherent and fully incoherent sweeps. This is the aim of the following description. For a fully coherent sweep, which is 100% identical to a highly chirped laser pulse, the minimum achievable pulse duration τ coh is given by the total sweep bandwidth and the time-bandwidth product (0.44 for a Gaussian envelope): To estimate the shortest pulse duration that can be achieved by compressing a fully incoherent wavelength-swept waveform, we assume a tunable optical bandpass filter with a spectral width Δ λ Filter where the filter passband is swept over a spectral range Δ λ sweep in a time τ sweep . The tuning speed is assumed to be constant: Here the ratio between filter bandwidth Δ λ Filter and tuning range Δ λ sweep defines the number of resolvable wavelengths n =Δ λ sweep /Δ λ Filter within the sweep. Note that in the case of tunable lasers with mode competition, the output can exhibit a more narrowband instantaneous linewidth Δ λ inst than the width of the filter Δ λ Filter . Therefore, in general, the number of resolvable wavelengths has to be defined as n =Δ λ sweep /Δ λ inst . The minimum pulse duration achievable by compressing fully incoherent wavelength sweeps is determined by two different limits (limit 1 and limit 2), which are discussed separately in the following. Depending on the sweep speed and the spectral filter width, either limit 1 or limit 2 is the dominant contribution. Limit 1, which arises as a direct consequence of wavelength sweeping, is the dominant contribution in the case of a sufficiently slow sweeping operation or a sufficiently wide filter. In this case, the resolvable spectral sections in the wavelength-swept waveform are equivalent to resolvable temporal sections. Consequently, we can define a switching time of τ switch = τ sweep / n , where τ switch is the time the filter needs to sweep over its bandwidth. As amplitude and phase of the optical waveform fluctuate randomly during each time interval τ switch , this, under given assumptions, is the shortest pulse duration that can be expected by compressing a wavelength sweep generated from an incoherent light source. Hence, the minimum achievable incoherent pulse width τ inc = τ switch is determined by the filter width (or the instantaneous linewidth) and the sweep speed: More narrowband filters and higher sweep speed will result in shorter pulses. However, there is an additional condition determining the minimum pulse duration. The time-bandwidth limit (limit 2) sets a lower boundary to the shortest pulse duration, and in incoherent swept sources the filter width Δ λ Filter or the instantaneous linewidth Δ λ inst determines this limit (in fully coherent sources it is the sweep width Δ λ sweep ). Limit 2 is the dominant contribution assuming a sufficiently high tuning speed (or sufficiently narrowband filter widths). In this case, we can estimate the minimum achievable pulse duration for a Gaussian shape at a centre wavelength of λ c and the speed of light c : In general, the minimum achievable pulse duration τ inc of fully incoherent swept sources can be obtained by convoluting both contributions (limit 1 and limit 2). Assuming Gaussian-shaped temporal windows ( τ inc is FWHM), the minimum pulse duration reads: Experimentally, fully incoherent swept sources can be realized by filtering temporally incoherent light, such as a thermal source or, in our case, spontaneous emission from an SOA. Such a source has been described in [36] and [37] . In such sources, the instantaneous linewidth Δ λ inst is always identical to the filter width. Instantaneous linewidth of the FDML laser Measuring the instantaneous linewidth Δ λ inst of a rapidly wavelength-swept light source is not trivial, especially as, at very high sweep speed, the values approach the time-bandwidth limit [35] . One approach, that is very common in swept source OCT, but yielding only an average value for the instantaneous spectrum (average over one sweep), is the following: the interference signal from a Michelson interferometer is acquired and a combined analysis of phase jitter and loss in fringe contrast using a Fourier transform is used to determine the coherence length, and with it the instantaneous spectrum. As the fringe frequency increases beyond our measurement bandwidth (1 GHz—Tektronix real-time oscilloscope type DPO 7104), for a very narrow instantaneous linewidth Δ λ inst , we cannot measure down to the −6 dB coherence roll-off, but only to ~−0.5 dB. Extrapolation of our data allows for a rough estimation of Δ λ inst to ~10 pm, which corresponds to ~1.2 GHz at 1,560 nm. This value is used in the diagram in Fig. 4b to estimate the level of coherence in the FDML sweep. How to cite this article : Eigenwillig, C. M. et al. Picosecond pulses from wavelength-swept continuous-wave Fourier domain mode-locked lasers. Nat. Commun. 4:1848 doi: 10.1038/ncomms2870 (2013).